Low-density three-dimensional foam using self-reinforced hybrid two-dimensional atomic layers Low-density nanostructured foams are often limited in applications due to their low mechanical and thermal stabilities. Here we report an approach of building the structural units of three-dimensional (3D) foams using hybrid two-dimensional (2D) atomic layers made of stacked graphene oxide layers reinforced with conformal hexagonal boron nitride (h-BN) platelets. The ultra-low density (1/400 times density of graphite) 3D porous structures are scalably synthesized using solution processing method. A layered 3D foam structure forms due to presence of h-BN and significant improvements in the mechanical properties are observed for the hybrid foam structures, over a range of temperatures, compared with pristine graphene oxide or reduced graphene oxide foams. It is found that domains of h-BN layers on the graphene oxide framework help to reinforce the 2D structural units, providing the observed improvement in mechanical integrity of the 3D foam structure. The intriguing architecture and properties of cellular solids in nature have inspired researchers to create their biomimetic replicas [1] , [2] . These man-made, low-density, highly porous materials called foams, exhibit novel physical properties compared with their bulk counterparts. Large specific area, high energy absorption at impact and outstanding strength to weight ratios make them ideal for catalysis, energy storage, damping and building structural components [3] , [4] , [5] . Creating three-dimensional (3D) structures using nanoscale elements allow tailoring of properties by integrating specific elements in favourable proportions [6] , [7] , [8] . Although a wide range of nano-sized elements in different dimensionalities can be used, the fascinating physical phenomena in materials at atomic layer thicknesses make two-dimensional (2D) materials such as graphene, boron nitride and transition metal dichalcogenides extremely attractive building blocks for macroscopic multilayer assemblies [9] , [10] , [11] . 3D frameworks can be built from these 2D materials by template assisted growth or self-assembly in solution by van der Waals forces or chemical cross-linking [12] , [13] , [14] . Building 3D interconnected structure from 2D materials is still in infancy stage and most of the previous reports are on graphene-based foams [15] , [16] , [17] , [18] , [19] . This is due to the excellent electrical, thermal and mechanical properties of graphene combined with the reactive edges that allows functionalization [20] , [21] , [22] , [23] . Nevertheless, compared with the explosion of work done on 2D graphene and graphene-based materials such as graphene oxide (GO), there have been only few reports about the 3D nanoengineered structures built from them. Both chemical vapour deposition and solution processing methods have been used in the past for developing 3D architecture of the above-mentioned materials [15] , [16] , [17] . The complex setup and poor scalability of chemical vapour deposition process make self-assembly in solution the ideal synthesis route for the bottom-up approach. The 3D structures formed by GO and graphene were predominantly open porous networks with no ordered stacking. The eventual freeze drying process for removing water from the macroporous networks were found to leave the nanoflakes forming the structural units crumbled and bent [24] . An adverse effect of this is conspicuous in the thermal and mechanical stabilities of the foams created for these units. For many practical applications, graphene nanocomposites are preferred for synergistic effects that allow controlled functionality. The heterostructures formed by atomic layer stacking of hexagonal boron nitride (BN) with graphene have led to very interesting optical, electronic and mechanical properties [25] , [26] , [27] , [28] , [29] . The chemical inertness, high mechanical strength and the ability to withstand extremely high temperature make BN an ideal material for building monolithic and composite 3D scaffolds [30] , [31] , [32] , [33] . BN exists in different crystalline forms of which hexagonal boron nitride (h-BN) is the most structurally compatible form and is an isomorph of graphene [34] , [35] . A good lattice matching is observed in their hybrids. The present study focuses on the effect of unique interaction between h-BN and graphene and the role of h-BN in generating and strengthening graphene-based 3D structures. In the current work, we report the formation of h-BN reinforced layered 3D stacks of GO with adjacent layers connected to each other through a porous network. The strong physical interactions between h-BN and GO resulted in fairly uniform distribution of h-BN platelets throughout the foam. The h-BN domain prevents the GO flakes from crumbling and binds them to form large plates. The layered restacking of these plates forms a unique ordered 3D structure. The mechanical and thermal stabilities were significantly enhanced compared to the random open porous networks of GO foams without h-BN. The complex and novel structural formation which leads to an improved mechanical performance are further corroborated using molecular dynamics (MD) simulation. The foam prepared using simple wet chemistry followed by lyophilization can easily acquire the shape of the container. This allows low cost and large-scale synthesis of these structures. Synthesis and characterization of GO-BN 3D hybrids It has been identified that the synthesis of elementary 2D building blocks and their combinational stacking will lead to the development of new solids with multifunctional properties [36] . In an earlier attempt, we have developed such an extended solid from h-BN and graphene, where a solution-based self-assembly lead to the formation of a new solid [24] . The solution mixing of GO and h-BN also forms similar solids and their difference in lateral size forms h-BN decorated GO sheets. The solution processing method for producing covalently interconnected GO sheets was used in making the GO-BN composite foams [17] . The mechanism of cross-linking of GO sheets is explained in our previous report [17] , where glutaraldehyde forms hemiacetal group with hydroxyl groups (-OH) in the adjacent GO sheets. The higher number of –OH groups in GO facilitates the cross-linking between adjacent sheets via aging (24 h), and the resultant solution is subjected to freeze drying process. An ultralow density (~5 mg cm −3 , that is, 1/400 times density of graphite) foam cast in the shape of the vial as shown in Fig. 1a was obtained after lyophilization. The foam is named GO-0.5BN where 0.5 stands for the weight fraction of h-BN in the composite. GO-0.5BN was viewed at different magnifications and different tilted projections using scanning electron microscope (SEM) as shown in Fig. 1b–f . The high-magnification image of the top layer shows ( Fig. 1b ) platelets of h-BN embedded in the layer. The low-magnification image Fig. 1d shows the several microns long 2D sheets of h-BN embedded GO with nanometre thickness stacked on top of each other. These layers are stacked on each other by a porous interconnected ( Fig. 1c ) film constituted by GO flakes joining perpendicular to the larger layer as shown in Fig. 1e–f . The plan view of interconnected film is shown in Fig. 2c . The high-magnification image of the region shown in Fig. 1e reveals the thickness of these films and their in-plane and out-of-plane cross-linking connection. The elevation view of these layers shows ( Fig. 1f ) clear junction to larger layer. The fine platelets are surrounded by a local strain distribution in the layer. A schematic of the 3D structure is shown in Fig. 1g . 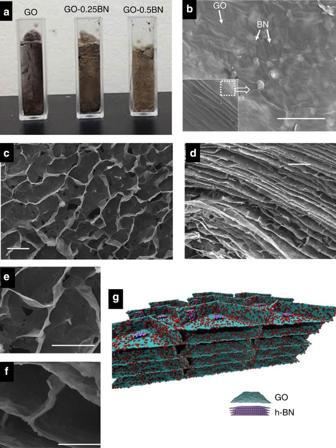Figure 1: Morphology of the 3D GO-BN Foam. (a) Photograph of GO foams with varying concentrations of h-BN. (b–f) SEM images showing the layered interconnected structure of GO-0.5BN. Different views show (b) h-BN embedded in GO and the low-magnification image in the inlay shows the presence of h-BN large in-plane connected layers of GO, scale bar, 2 μm; (c) interconnecting porous network between the layers, scale bar, 10 μm; (d) low-magnification image showing layers stacked to form 3D structure, scale bar, 100 μm; (e,f) the 3D connection between layers in different magnifications. Scale bars, (e) 2 μm, (f) 100 nm. (g) Proposed schematic for GO-0.5BN foam based on SEM observations. Figure 1: Morphology of the 3D GO-BN Foam. ( a ) Photograph of GO foams with varying concentrations of h-BN. ( b – f ) SEM images showing the layered interconnected structure of GO-0.5BN. Different views show ( b ) h-BN embedded in GO and the low-magnification image in the inlay shows the presence of h-BN large in-plane connected layers of GO, scale bar, 2 μm; ( c ) interconnecting porous network between the layers, scale bar, 10 μm; ( d ) low-magnification image showing layers stacked to form 3D structure, scale bar, 100 μm; ( e , f ) the 3D connection between layers in different magnifications. Scale bars, ( e ) 2 μm, ( f ) 100 nm. ( g ) Proposed schematic for GO-0.5BN foam based on SEM observations. 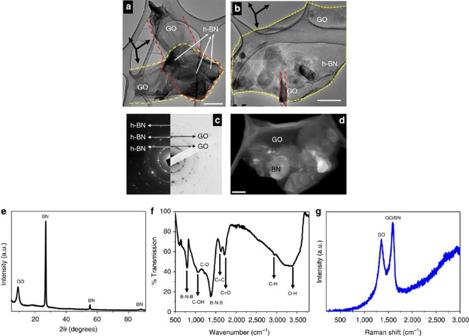Figure 2: Material characterization of GO-0.5BN. (a–d) TEM analysis of h-BN embedded GO sheets constituting the fundamental units of the foam revealing (a) two adjoining GO sheets with h-BN providing support at the point of contact, scale bar, 0.5 μm; (b) h-BN embedded in flat GO sheet and 3D structure originating from perpendicularly attached GO flake (marked in red dotted line), scale bar, 0.5 μm; (c) diffraction pattern corresponding to the hexagonal lattices of h-BN (multilayered) and GO; (d) HADDF showing smaller-sized multilayered h-BN distributed along GO, scale bar, 200 nm; (e) XRD showing GO peak at ~10 degrees and h-BN peak at ~27 degrees. (f) FTIR showing different bond vibrations in GO and h-BN, (g) Raman spectra showing the D band for GO and G band for GO and h-BN. a.u., arbitrary unit., HADDF, high angle annular dark field. Full size image Figure 2: Material characterization of GO-0.5BN. ( a – d ) TEM analysis of h-BN embedded GO sheets constituting the fundamental units of the foam revealing ( a ) two adjoining GO sheets with h-BN providing support at the point of contact, scale bar, 0.5 μm; ( b ) h-BN embedded in flat GO sheet and 3D structure originating from perpendicularly attached GO flake (marked in red dotted line), scale bar, 0.5 μm; ( c ) diffraction pattern corresponding to the hexagonal lattices of h-BN (multilayered) and GO; ( d ) HADDF showing smaller-sized multilayered h-BN distributed along GO, scale bar, 200 nm; ( e ) XRD showing GO peak at ~10 degrees and h-BN peak at ~27 degrees. ( f ) FTIR showing different bond vibrations in GO and h-BN, ( g ) Raman spectra showing the D band for GO and G band for GO and h-BN. a.u., arbitrary unit., HADDF, high angle annular dark field. Full size image Field emission gun transmission electron microscopy (TEM) has been extensively used for observing the basic 2D building blocks followed by the 3D structure. The size and structural analysis of initial raw 2D nanosheet of GO and h-BN performed using TEM is shown in Supplementary Fig. 1 . It shows a larger GO nanosheet and smaller-sized h-BN flakes. Several images from different samples has been used to determine the mean sheet dimension which was found to be micron size GO and ~400 nm size h-BN nanosheet with an average of two-layer thickness. To understand the role of h-BN in structure formation, a detailed TEM of GO without h-BN and with two fractions of h-BN has been performed. A representative low-magnification transmission electron microscope (TEM) images show h-BN embedded in the large GO flakes as shown in Fig. 2a . The presence of h-BN in multilayers possibly resulted from inherent hydrophobicity and high concentration of solution used for lyophilization. Figure 2a shows h-BN providing support to two adjoining few-layered GO flakes and the red marked area in Fig. 2b has GO perpendicularly attached to a horizontal flake, which shows the origin of the 3D architecture. The selected area electron diffraction pattern shown in Fig. 2c confirms the hexagonal lattices of h-BN and graphene. High angle annular dark field micrograph shown in Fig. 2d reveals that multilayered h-BN is distributed in GO. The sharp edges of GO layer are seen where there is high concentration of h-BN but the absence of h-BN results in the bending of other edge areas. It clearly reveals a high impact of h-BN on the morphology of GO sheet. The bulk phase and structural characterization of these foams were performed using X-ray diffraction (XRD), Raman spectroscopy and Fourier transform infrared spectroscopy (FTIR). XRD shown in Fig. 2e reveals a peak at 2θ=10 degrees for GO (001) corresponding to an interlayer spacing of 8.8 Å and for h-BN (002) at 2θ=27 degrees corresponding to a lattice constant of 3.29 Å. FTIR was used to detect the different bonds and functionalities present in the sample ( Fig. 2f ). The spectrum shows different functional groups of GO at ~3,420 cm −1 (O–H stretching vibrations), ~2,950 (C–H stretching vibrations), ~1,720 cm −1 (C=O stretching vibrations), ~1,210 cm −1 (C–OH stretching vibrations) and ~1,060 cm −1 (C–O stretching vibrations). In addition to these, the skeletal vibrations from unoxidized C=C bonds was seen at ~1,620 cm −1 . The B-N-B in-plane vibrations (E 1u mode) for h-BN was assigned to ~1,370 cm −1 and the out-of-the-plane B-N-B vibrations (A 2u mode) to ~800 cm −1 . All the above characterization also clearly confirms absence of any other impurity. Raman spectrum shows the G band at ~1,580 cm −1 and D band at ~1,340 cm −1 ( Fig. 2g ). The G band is common to both GO and h-BN, which arises from the first-order scattering of E 2g mode and the D band is from the basal plane defects created by the presence of functional groups in GO. To understand the role of BN in forming these 3D stacked structures, GO (GO-0.0BN) and GO with 25% h-BN (GO-0.25BN) were also synthesized by keeping the overall concentration and procedure same as in GO-0.5BN. Although GO-0.0BN has interconnected network as that of GO-0.5BN, the stacked structure with micron-sized 2D layer is absent. The high-magnification SEM image in Fig. 3a shows GO-0.0BN that consists of interconnected GO layers and resembles the structure in Fig. 1c , which is the porous mesh between the layers in GO-0.5BN. The GO without BN are bent from edges as clear from both low-magnification and high-magnification-images. The high-magnification top view of the GO-0.25BN ( Fig. 3b ) shows very similar structure as that of GO-0.5BN with fewer fractions of h-BN platelets on top. This reaffirms our assumption that h-BN is the key element in obtaining the stacked 3D architecture. The morphology of these structures is further confirmed using low-magnification TEM images shown in Fig. 3c,d . The TEM image of GO shows wrinkled and folded sheets ( Fig. 3c ) in contrast to the flat sheets seen in samples with h-BN ( Fig. 3d ). The curling was only found at the edges of the sheets in GO-0.25BN where there is minimum concentration of h-BN platelets (marked by arrow). 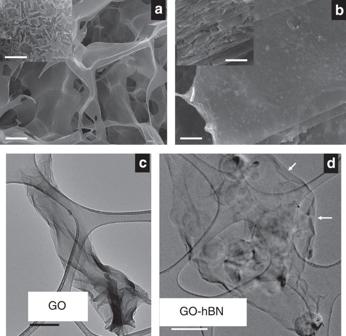Figure 3: SEM and TEM characterization of GO-0.0BN and GO-0.25BN. (a) SEM image of GO-0.0BN showing the interconnected porous structure but absence of large layers. Scale bars, 20 μm, (inlay) 50 μm. (b) SEM image of GO-0.25 which shows large layers similar to GO-0.5BN. Scale bars, 20 μm, (inlay) 50 μm. (c) TEM image of GO-0.0BN showing wrinkled sheets of GO as there is no h-BN present on it. Scale bars 0.5 μm (d) TEM image of GO-0.25BN with flat GO sheets and curling only on the edges where there is less concentration of h-BN. Scale bars 20 μm, (inlay) 50 μm. Figure 3: SEM and TEM characterization of GO-0.0BN and GO-0.25BN. ( a ) SEM image of GO-0.0BN showing the interconnected porous structure but absence of large layers. Scale bars, 20 μm, (inlay) 50 μm. ( b ) SEM image of GO-0.25 which shows large layers similar to GO-0.5BN. Scale bars, 20 μm, (inlay) 50 μm. ( c ) TEM image of GO-0.0BN showing wrinkled sheets of GO as there is no h-BN present on it. Scale bars 0.5 μm ( d ) TEM image of GO-0.25BN with flat GO sheets and curling only on the edges where there is less concentration of h-BN. Scale bars 20 μm, (inlay) 50 μm. Full size image Mechanical testing The ultralow density GO-0.5BN foam shows unique sponge behaviour. The mechanical testing of the foams was performed using controlled strain and load experiments using dynamical mechanical analyser. In the controlled strain experiments, the foams were subjected to three different strains S 1 (0.5%), S 2 (1%) and S 3 (2%) applied in sequence and the stiffness was recorded as a function of time. In the first step, strain is applied for 30 min, released and then re-applied again. The same process is followed subsequently for other strains and performed on all the three samples. GO-0.0BN shows a constant stiffness at S 1 strain and at higher strain, the stiffness drops drastically as shown in Fig. 4a . This may be due to permanent deformation in the sample. On the other hand GO-0.5BN ( Fig. 4b ) and GO-0.25BN ( Supplementary Fig. 2 ) reveals a different behaviour. GO-0.5BN shows an increase in stiffness as time increases. The behaviour remains same in next cycles of strains as well. GO-0.25BN also exhibits a similar behaviour and is shown in Supplementary Fig. 2 . The samples were further subjected to load control experiments. 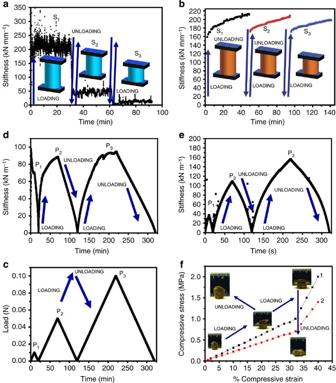Figure 4: Controlled strain/load experiments and compression testing. (a,b) Controlled strain experiments with three different strains S1(0.5%), S2(1%) and S3(2%) applied in sequence and stiffness monitored for (a) GO-0.0BN where a drastic drop in the stiffness is observed after S2is applied due to permanent deformation, (b) GO-0.5BN where the stiffness is maintained during different cycles. (c–e) Controlled load experiment where three different maximum loads P1, P2and P3were applied as shown inc, the loading/unloading cycles ond, GO-0.0BN where a compression is observed in the lowest load and permanent deformation in subsequent loads, (e) GO-0.5BN where stiffness does not decrease during different loads, exhibiting complete recovery. (f) Compression test results on Instron showing a linear increase in stress until 35% strain; the photographs show GO-0.5BN taking the load of 2.5 g and 5 g and resuming the original shape after unloading. Figure 4c–e shows loading and unloading cycles applied in GO-0.0BN and GO-0.5BN. Three different maximum loads P 1 , P 2 and P 3 were applied and the stiffness was measured during this process. For GO-0.0BN, in lowest load, the load and unload curve shows a compression; that is, a drop in stiffness as seen in strain control test. On further loading, it loads but rapidly unloads with a drastic drop in stiffness. On higher loading cycle, the maximum stiffness remains same but the break in stiffness shows a clean fracture in the foam. On the other hand GO-0.5BN shows similar behaviour of stiffness in loading/unloading cycle and can be interpreted as complete recovery without any permanent deformation. GO-0.5BN shows remarkable recovery and is tested using Instron at a strain rate of 10 −3 s −1 . It shows a linear increase in stress till 30–35% after which it starts compacting on further load as seen in Fig. 4f . The same behaviour is observed for GO-0.25BN. The foams were loaded with weight of 2.5 g (United States penny coin was used as the weight) and it was found to compress 20% and after removing the load, it returned back to its original shape. On higher load of 5 g (two pennies placed on top of each other), it deformed permanently, but still did not fracture. The deformed GO-0.0BN and GO-0.5BN samples were observed under SEM. 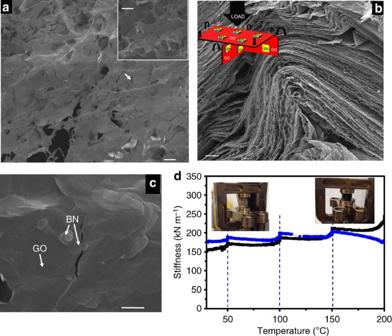Figure 5: Analysis of mechanical deformation in GO-0.0BN and GO-0.5BN and high temperature compression testing. (a) Low-magnification SEM revealing cracking along GO sheets and also at the junctions; high magnification is shown in inlay confirms the inferences. Scale bars, 10 μm, (inlay) 1 μm. (b) Low-magnification SEM of GO-0.5BN showing the layers bending rather than cracking and the alignment of load along the structure is shown in the schematic (inlay). Scale bar, 50 μm. (c) High-magnification SEM showing small crack along the large layer where h-BN prevents it from propagating. Scale bar, 50 nm. (d) Compression testing at high temperature on GO-0.25BN and GO-0.5BN showing stiffness is stable to temperature as high as 200 °C. Figure 5a shows low-magnification image of GO-0.0BN with high-magnification image in inlay. There are multiple cracks passing across the GO sheet as well as at the junctions formed by cross-linking. Several small cracks are observed near the main crack as marked by arrow. This implies that the bonds between GO are not strong enough to overcome the strain and tends to break apart resulting in poor mechanical behaviour. Figure 5b shows low-magnification SEM image of GO-0.5BN after deformation. The layered structure is still present but the compression creates bending of these layers. The distribution of load by bending of layers prevents the whole structure from breaking. The load distribution in single entity of the 3D structure is shown as inlay. Infrequent small cracks are created along the layers (as seen in high-magnification SEM in Fig. 5c ) due to some tensile stress created in regions where there is no significant bending. But it is observed that the cracks are hindered when it encounters h-BN platelets. The bending of layers and the prevention of crack propagation along layers coactively contribute to the mechanical strength of GO-0.5BN. The effect on mechanical behaviour due to temperature variation is tested in GO-0.5BN and GO-0.25BN where both are subjected to high temperature mechanical testing and the stiffness was stable even at 200 °C as shown in Fig. 5d . Only small weight fraction loss in that temperature range was seen in thermogravimetric analysis as shown in Supplementary Fig. 3 . The weight loss in the case of higher h-BN concentration shows lower weight loss which is expected as h-BN has a very high temperature stability. The SEM of GO-0.5BN ( Supplementary Fig. 4 ) tested at high temperature shows that the 3D morphology remains still intact and confirms its structural stability. Figure 4: Controlled strain/load experiments and compression testing. ( a , b ) Controlled strain experiments with three different strains S 1 (0.5%), S 2 (1%) and S 3 (2%) applied in sequence and stiffness monitored for ( a ) GO-0.0BN where a drastic drop in the stiffness is observed after S 2 is applied due to permanent deformation, ( b ) GO-0.5BN where the stiffness is maintained during different cycles. ( c – e ) Controlled load experiment where three different maximum loads P 1 , P 2 and P 3 were applied as shown in c , the loading/unloading cycles on d , GO-0.0BN where a compression is observed in the lowest load and permanent deformation in subsequent loads, ( e ) GO-0.5BN where stiffness does not decrease during different loads, exhibiting complete recovery. ( f ) Compression test results on Instron showing a linear increase in stress until 35% strain; the photographs show GO-0.5BN taking the load of 2.5 g and 5 g and resuming the original shape after unloading. Full size image Figure 5: Analysis of mechanical deformation in GO-0.0BN and GO-0.5BN and high temperature compression testing. ( a ) Low-magnification SEM revealing cracking along GO sheets and also at the junctions; high magnification is shown in inlay confirms the inferences. Scale bars, 10 μm, (inlay) 1 μm. ( b ) Low-magnification SEM of GO-0.5BN showing the layers bending rather than cracking and the alignment of load along the structure is shown in the schematic (inlay). Scale bar, 50 μm. ( c ) High-magnification SEM showing small crack along the large layer where h-BN prevents it from propagating. Scale bar, 50 nm. ( d ) Compression testing at high temperature on GO-0.25BN and GO-0.5BN showing stiffness is stable to temperature as high as 200 °C. Full size image Molecular dynamics simulation of 2D building blocks The innovative and complex 3D structure formation due to h-BN and the influence of h-BN in mechanical behaviour of GO sheets were studied using fully atomistic simulations. A comparative simulation between GO sheet with and without h-BN has been performed. For close resemblance with experimental work, we have maintained the same ratio of dimension of the two nanosheets. It is important to note that the 3D structure consists of 2D sheets which undergo tension in one direction and results compression in the other direction. Keeping above in mind we have applied tension in one direction and compared naked GO and GO with h-BN flakes. Stretching process was simulated at temperature of 300 K until the cracking point and due to that a reactive force field, ReaxFF [37] , was chosen for these simulations. ReaxFF is similar to standard nonreactive force fields such as MM3 with the difference that it can describe bond formation and dissociation (making or breaking bonds) as a function of bond order values. For GO-BN, a finite h-BN was placed in the middle/top of the semi-infinite GO membranes (see Fig. 6 ). The strain was generated by gradual increase of the unit cell value along periodic direction. The stress was calculated by computing the forces on each atom and then obtaining the stress tensor. From this tensor, we calculated a quantity known as von Mises stress, the second invariant of the deviatoric stress tensor, which is related to the distortion state of the system. Von Mises stress provides very helpful information on the fracturing processes as it is possible to visualize the time evolution of the local stress. This methodology has been successfully used to investigate the mechanical failure of carbon-based nano structures such as graphene and carbon nanotubes and also h-BN structures [38] , [39] , [40] . 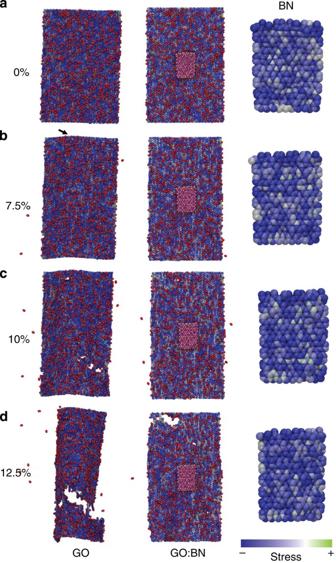Figure 6: MD simulation results of mechanical behaviour of naked GO sheet and GO sheet partially covered with h-BN (GO:BN) on application of different strains. (a) 0% showing the original shapes of GO and GO:BN, (b) 7.5% where stress is distributed uniformly along GO and there is an out-of-plane distortion; there is localized stress around h-BN bordering along periodic direction but no distortion allowed by h-BN, (c) 10% where stress distribution causes GO to break thereby provoking out-of-plane distortion; in GO:BN, the small crack in GO sheet is not allowed to propagate, (d) 12.5% where high-order cracking and crumbling is observed in GO; in GO:BN the stress distributed along periodic direction leads to a crack along the edges of GO sheet away from h-BN and no crumbling is observed. Figure 6: MD simulation results of mechanical behaviour of naked GO sheet and GO sheet partially covered with h-BN (GO:BN) on application of different strains. ( a ) 0% showing the original shapes of GO and GO:BN, ( b ) 7.5% where stress is distributed uniformly along GO and there is an out-of-plane distortion; there is localized stress around h-BN bordering along periodic direction but no distortion allowed by h-BN, ( c ) 10% where stress distribution causes GO to break thereby provoking out-of-plane distortion; in GO:BN, the small crack in GO sheet is not allowed to propagate, ( d ) 12.5% where high-order cracking and crumbling is observed in GO; in GO:BN the stress distributed along periodic direction leads to a crack along the edges of GO sheet away from h-BN and no crumbling is observed. Full size image As there is a significant strain induced in the foam during processing and testing, the simulations give us an insight into the structural formation and mechanical stability of the h-BN reinforced GO foam. The snapshots of stretching process with stress distributions for naked GO flake and GO partially covered with h-BN flake at different strains are shown in Fig. 6 . First row of Fig. 6 shows GO and GO with h-BN at initial stage (0% strain). Note that the interaction between h-BN and GO produces a more stressed structure than naked GO. When the strain (see 7.5% strained), is continuously applied, the resulting stress is distributed uniformly through GO, which presents an out-of-plane distortion (shown by arrow). On the other hand, though small, for same strain, GO-BN structure concentrates stress in localized regions across area of BN and border along periodic direction and no distortion is allowed by h-BN coverage, which explains our TEM observation. Because of uniform stress distribution, at 10% strain, naked GO starts to break from edges close to the membrane centre. This cracking provokes a high out-of-plane distortion in GO sheet. As the stress in GO-BN is more concentrated on borders along periodic direction, the same cracking area in GO remains intact with only presence of a small hole that does not propagate. An extensive cracking is observed in GO sheets without h-BN at ~12.5% strain, where the flake starts to break apart. Only at that strain of ~12.5%, a cracking occurs for GO-BN. For this case, the stress distributed on borders along periodic directions induces a parallel cracking at the edges away from h-BN without any bending or buckling, thereby providing more structural stability. These results are in agreement with the inferences from SEM and TEM images. From the simulation, it is possible to highlight two main effects of h-BN coverage. The first one is related to the changes in stress distribution. The interaction between h-BN and GO complicates the stress distribution along structure, which concentrates in the region immediately close to where strain is generated (border along periodic direction). In addition, h-BN also alters the out-of-plane deformation of structure. These effects induce a completely different process of stretching and consequently different cracking patterns for pristine GO and GO-BN as we observe from Fig. 6 . To further investigate the mechanical stability, the effect of h-BN on single out-of-the-plane GO sheet (which is the GO sheet in the porous network as indicated in Supplementary Fig. 5a ) during compression was also studied and is shown in Supplementary Fig. 5b,c . Significant bending is induced in GO sheet in naked GO, but in GO-BN the bending is restricted to regions where h-BN is not present. An increased threshold fracture limit and more efficient stress accumulation and dissipation is observed on GO with h-BN compared with naked GO flake. During compression, deformation occurs on h-BN and this in turn minimizes bending of the large GO flake. Hence in naked GO, buckling can occur at lower stress leading to early fracture. The bending/buckling gives rise to high stress concentration at the bent edge leading the local stress to cross the critical stress (fracture value). These results indicate the superior mechanical behaviour in h-BN reinforced GO flakes at 2D level and it is very critical in the overall structural formation and mechanical performance of the entire 3D structure. Unlike the hydrogel/aerogel structures formed from graphene-based materials reported earlier, the novel architecture reported here has macro-sized layers of conjoined GO sheets orderly stacked with the out-of-plane mesh completing the 3D framework. The innovation and improvement in mechanical properties and stabilities lie in the structure of the 3D foam. The comparative study between GO only and h-BN reinforced GO foams clearly reveals that h-BN in GO sheet has very important role in the formation of 3D layered network structure. First of all, the atomic level interactions between h-BN and GO were found to aid the formation of nearly flat flexible layers, which is further observed in our MD simulation. The higher stiffness of h-BN does not allow the GO sheet to bend due to in-plane lateral stress. The presence of h-BN maintains the GO sheet flat and there are wrinkles only in few areas. This results in increased van der Waals forces between similar sheets face to face and as the sheets are dispersed in water and not aligned, they stack together partially overlapping with each other resulting in formation of large layers. The cross-linking between GO sheets also aids the formation of layers and is considered accountable for the 3D connection between the layers. The spacing between the layers is attributed to the mutual interaction of van der Waals forces and electrostatic repulsions due to the ionized carboxylic and phenol hydroxyl groups in GO. However in the absence of h-BN, the sheets are wrinkled and the formation of large layer is not possible and they form an interconnected porous network due to the crosslinking by GAD and Resorcinol. The TEM and SEM data show multilayered h-BN preventing the GO sheets from breaking by significantly reducing the crack propagation from the strain induced during lyophilization. The HRTEM image showing dislocation reveals role of h-BN in GO sheet in distribution of stress ( Supplementary Fig. 6 ). The stress generated during the process of freeze drying is transferred from GO sheet to a multi fold higher stiff h-BN nanosheet. The dislocation at the interface of GO and h-BN confirms the above phenomena. The same is also observed in our MD simulation results. MD simulation is consistent with the electron microscopy results and the drastic change in the structure formation in the presence and absence of h-BN is attributed to the difference in stress distribution in the two cases. While the uniform stress distribution in GO results in the in-plane cracking and out-of-plane distortion, the complex stress distribution in h-BN-covered GO restrains the crack from propagating. These results elucidate the layered assembly and the enhanced mechanical stability of the GO-BN foams. As discussed in the previous section, the foam consists of two types of 2D sheets which align in two directions to loading. The schematic of the alignment of loading to the sheets is shown as inlay in Fig. 5c . In this type of foam structure consisting of high stiffness and high modulus GO-h-BN sheet with high fracture toughness, the top sheet transfers the load to perpendicular aligned sheet and undergoes tension at other places. The sheet aligned parallel to load direction undergoes compression bending due to small thickness. The large layers do not fracture even at much higher load due to the presence of h-BN mitigating the cracks ( Fig. 5c ). Also the stress is localized near h-BN platelets (also shown in Fig. 3g ) and gets relaxed and transmitted through the sheet during unloading. Changing loading direction shows a change in properties which proves anisotropy of the 3D foam behaviour ( Supplementary Fig. 7 ). On the other hand, the randomly oriented GO sheet foam without h-BN however shows similar stiffness but fails after first loading. In summary, a unique reinforcement effect of h-BN was demonstrated and investigated in GO-based ultralow density 3D hybrids. Excellent elastic behaviour was demonstrated by the GO-BN foam up to a strain of ~40%. The mechanical stiffness was unchanged and the structural integrity was retained even at higher temperatures. The high mechanical and thermal stabilities of the foam overcome the major limitations associated with conventional nanoengineered foams. The simple processing and scalability of the foams enable developing them in desired shapes and sizes. Synthesis of GO-BN foams GO was prepared from graphite powder (45 μm, 99.99%, SP-1 Bay Carbon) using improved Hummer’s method reported elsewhere [41] . Liquid exfoliation method was followed for synthesizing few-layered h-BN flakes [42] . The starting material used was h-BN powder (1 μm, 98%) from Sigma Aldrich. Dimethyl formamide (DMF, room temperature surface tension ~37 mN m −1 ) was obtained from Sigma Aldrich and used as the exfoliation fluid medium. The micron-sized h-BN powder was added to the container batches with DMF. Subsequently, the prepared solution was extensively sonicated (~5 h) in a Branson 5510 water bath sonicator, keeping the temperature of the water bath constant (room temperature ~300 K). After sonication, the solution was centrifuged with a Thermo Fisher Scientific sorvall biofuge stratos centrifuge for 30 min at 1,500 r.p.m. The whitish supernatant (top part) is decanted and was vacuum filtered, using a Sartorious PTFE—filter membrane with a pore size of 0.2 μm. After this process, 2D h-BN nanosheets (~500 nm by 500 nm, approximatelyfive layers in thickness) were obtained [33] . The h-BN nanosheets were washed twice with water, ethanol and chloroform to remove any residual DMF and the dried material was then scraped off from the filter paper. Equal weight amounts of GO and h-BN were separately sonicated in deionized water for 30 min and mixed together to make a concentration of 10 mg ml −1 . Resorcinol (0.25 mg ml −1 ), glutaraldedhyde (2 μl ml −1 ) and a very small amount (~0.1 mg) of sodium tetraborate decahydrate was added to the GO-BN dispersion and sonicated for 2 h. The solution was then lyophilized in a bench-top freeze dryer (MillRock Technology) for 48 h. Material characterization and mechanical testing Raman spectroscopy was done using Renishaw in Via Raman Microscope at laser excitation of 514.5 nm. Nicolet FTIR Infrared Microscope was used for performing FTIR on the sample for studying the chemical bonds present. The morphology of the samples was observed using FEI Quanta 400 scanning electron microscope under high vacuum at 10 kV. A 10-nm thick gold film was sputtered on the sample before imaging for reducing the charging effects from h-BN. TEM images and diffraction patterns were taken using JEOL 2100 field emission gun transmission electron microscope. For preparing the TEM samples, small pieces were broken from the foams and bath sonicated in isopropyl alcohol for 30 min. A few drops were then cast onto the holy-carbon grids and allowed to dry in vacuum. The TEM samples were then left under vacuum overnight. Q800 dynamic mechanical analysis was employed for performing mechanical test on the samples from room temperature up to 200 °C. Compressive stress versus strain curve was obtained from Instron universal testing machine. Simulation All calculations were carried out using the reactive force field ReaxFF [37] . This forcefield was parameterized using density functional theory calculations and, through bond length/bond order relationship, it can handle chemical reactions. The average deviation between ReaxFF heat of formation value and the experimental one is 2.8 and 2.9 kcal mol −1 for nonconjugated and conjugated systems, respectively. Similarly to standard nonreactive force fields, ReaxFF divides the system energy into partial energy contributions associated with terms such as: valence angle bending, bond stretching as well as nonbonded Coulomb and van der Waals interactions [37] . The main difference, however, is that ReaxFF can make and break bonds as a function of bond order values. In this way, the system energy for ReaxFF is composed by: where E bond is the bond energy, E over is over-coordination, under-coordination is E under , valency energy is E val , energy penalty for handling atoms with two double bonds is E pen , E tors is torsion energy, conjugated bond energies is E conj , van der Waals energy is E vdWaals and Coulomb energy is E coulomb . For better description of reactivity in the simulations, all bond orders were calculated and charge effects were taken into account in electronegativity equalization method approach [43] . For the stretching process and stress analysis, our system was composed by semi-infinite GO strips, generated by random distributions of oxygen atoms into graphene membranes. System temperatures were set to 300 K and controlled by a Nose–Hoover thermostat imposing a canonical ensemble with constant number of atoms, temperature and volume (NVT ensemble) as implemented on large-scale atomic/molecular massively parallel simulator [44] . Time-steps of 0.05 fs were used and a constant strain rate of 10 −6 fs −1 was continuously implemented during the whole simulation until the mechanical rupture. Stress values are obtained calculating the force per atom at each step of simulation and then subtracted from the hydrostatic components to obtain the deviatoric stress and one of its invariants, the so-called von Mises stress. von Mises stress describes the distortion stress state and provide relevant information for the analysis of fracture mechanisms. How to cite this article: Vinod, S. et al. Low-density three-dimensional foam using self-reinforced hybrid two-dimensional atomic layers. Nat. Commun. 5:4541 doi: 10.1038/ncomms5541 (2014).